The molecular origin of high DNA-repair efficiency by photolyase The primary dynamics in photomachinery such as charge separation in photosynthesis and bond isomerization in sensory photoreceptor are typically ultrafast to accelerate functional dynamics and avoid energy dissipation. The same is also true for the DNA repair enzyme, photolyase. However, it is not known how the photoinduced step is optimized in photolyase to attain maximum efficiency. Here, we analyse the primary reaction steps of repair of ultraviolet-damaged DNA by photolyase using femtosecond spectroscopy. With systematic mutations of the amino acids involved in binding of the flavin cofactor and the cyclobutane pyrimidine dimer substrate, we report our direct deconvolution of the catalytic dynamics with three electron-transfer and two bond-breaking elementary steps and thus the fine tuning of the biological repair function for optimal efficiency. We found that the maximum repair efficiency is not enhanced by the ultrafast photoinduced process but achieved by the synergistic optimization of all steps in the complex repair reaction. Photochemical machines in nature are powered by sunlight to execute important biological functions such as photosynthesis for light energy conversion to chemical energy and photosensory function for signal transduction [1] , [2] , [3] , [4] , [5] , [6] . To reach high biological efficiency, the initial photoinduced dynamics are usually ultrafast to quickly funnel excitation energy into the functional coordinate(s) and avoid futile energy dissipation into the environment [2] , [3] , [4] . In addition to photosynthesis and photosignalling, blue light energy is used as a co-substrate for repairing DNA damage by photolyase with high quantum yield [7] , [8] . The photoenzyme performs biotransformation with multiple elementary chemical steps [9] , [10] , and at present it is not known whether the initial ultrafast photoinduced process is the determinant of high efficiency. Thus, a key question in photolyase research is how the enzyme optimizes elementary chemical reactions to achieve the high efficiency and the role of the rate of the initial photoinduced process in achieving high quantum yield. We recently mapped out the entire dynamics of DNA repair with six elementary reactions using femtosecond spectroscopy to follow the complete functional evolution ( Fig. 1a ) [11] , [12] , [13] , [14] . We observed two consecutive competitions of these elementary steps that make key contributions to the final repair efficiency: the first one is the forward electron transfer (ET, τ FET ) from the excited cofactor flavin (FADH − *) to substrate thymine dimer (T<>T), the major UV-induced DNA photoproduct [15] , against the deactivation process ( τ LT ), leading to the first-branching quantum yield Φ FET of 0.85. The second is the ultrafast splitting of the C5-C5′ and the C6-C6′ bonds ( τ SP2 ) relative to the futile back electron transfer ( τ BET ) without repair, resulting in the second-branching quantum yield Φ SP2 =0.96 ( Fig. 1a ). The overall repair efficiency (Φ T ) is the product of the two quantum yields and thus is as high as 0.82. 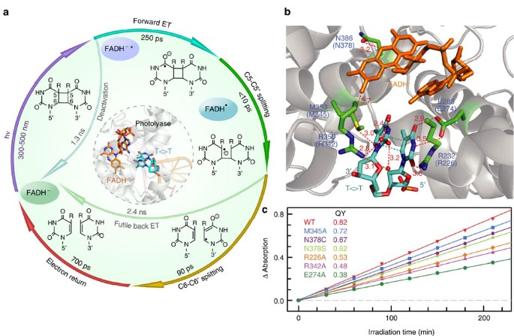Figure 1: Repair photocycle of ultraviolet-damaged DNA byE.coliphotolyase and the key functional residues in the active site with corresponding repair quantum yields. (a) The repair photocycle of UV-damaged DNA (thymine dimer) by photolyase with six elementary steps including one deactivation, three electron transfer and two bond-breaking reactions. Two competing processes with four main steps reduce the overall repair quantum efficiency. (b) Local structure at the active site with five critical residues (green), the cofactor flavin (orange) and substrate thymine dimer (cyan). The mutants of each of the five residues were examined for their contributions to the modulation of repair efficiency. Note the active site enzyme–substrate contacts are based onA. nidulansphotolyase-substrate co-crystal structure. The numbers in parenthesis indicate the corresponding residues inE. coliphotolyase. (c) Repair kinetics and repair quantum yields (QY) of wild-type photolyase and the six mutants analysed in this study. Figure 1: Repair photocycle of ultraviolet-damaged DNA by E.coli photolyase and the key functional residues in the active site with corresponding repair quantum yields. ( a ) The repair photocycle of UV-damaged DNA (thymine dimer) by photolyase with six elementary steps including one deactivation, three electron transfer and two bond-breaking reactions. Two competing processes with four main steps reduce the overall repair quantum efficiency. ( b ) Local structure at the active site with five critical residues (green), the cofactor flavin (orange) and substrate thymine dimer (cyan). The mutants of each of the five residues were examined for their contributions to the modulation of repair efficiency. Note the active site enzyme–substrate contacts are based on A. nidulans photolyase-substrate co-crystal structure. The numbers in parenthesis indicate the corresponding residues in E. coli photolyase. ( c ) Repair kinetics and repair quantum yields (QY) of wild-type photolyase and the six mutants analysed in this study. Full size image To understand how the enzyme achieves this high quantum efficiency, we use an oligonucleotide substrate containing cyclobutane thymine dimer (T<>T) and examine the contributions of the amino acids involved in the binding of cofactor (FADH − ) and substrate (cyclobutane pyrimidine dimer in DNA) to catalysis by using mutant enzymes that affect cofactor and substrate interactions as well as activate site dynamics that tune each elementary step in this multi-step catalytic reaction. We reveal that the maximal repair efficiency results from the overall synergy of all elementary steps. Oligonucleotide substrate and critical active-site mutants Previously, we investigated functional dynamics of photolyase by using di-pyrimidine cyclobutane dimers of various compositions and ultrafast spectroscopy and found that the enzyme repairs cyclobutane dimers with high quantum yield. To gain further insight into the contributions of various factors in the active site to catalytic efficiency in this study we used an oligonucleotide substrate and mutant forms of the enzyme that affect either the redox properties of the flavin or the properties of the substrate with following considerations. At the binding pocket of the substrate, salt bridges and hydrogen bonds are formed between the T<>T dimer and amino-acid residues: protonated E274 could form two hydrogen bonds with N3 and O4 of the 5′-thymine; R226 has both electrostatic interaction and hydrogen bond with 5′-thymine; R342 interacts with 3′-thymine not only through salt bridge but also through the water network. These hydrophilic interactions could disperse the excessive electron density and help stabilize the generated radical anion of the dimer after electron injection from FADH − *. Thus, the mutations of these binding-site residues would reduce the stabilization and lead to the decrease in the reduction potential of T<>T/ T<>T · − . As these mutations do not affect the reduction potential of the flavin cofactor, the free energy ( ) becomes less negative than that of the wild type. On the flavin cofactor side, N378 is opposite to the N5 position of flavin, and its side carbonyl group forms a hydrogen bond with the N(5)H group of FADH · or FADH − . Destroying the interaction would abolish the ability of photolyase to stabilize the FADH · radical [16] . These five critical residues at the active site that were studied are shown in Fig. 1b : N378 near the cofactor forms a hydrogen bond with the N5 atom of flavin, M345 is in the middle between the flavin cofactor and 3′ base of the substrate, and E274, R226 and R342 are around the substrate with the former two residues having hydrogen bonding with the 5′ base and the latter one forming a hydrogen-bond network with water molecules and the 3′ base [17] , [18] . We found that N378 mutated to serine (S) or cysteine (C) was necessary to obtain stable proteins, for the other four residues we used an alanine (A) scanning mutagenesis. Figure 1c shows our measurement of the total repair quantum yields of these six mutants, which ranges from 0.38 to 0.72, with the wild type (WT) having the highest repair efficiency of 0.82. Ultrafast electron injection and electron return To understand how each mutation modulates the elementary steps in catalysis, we mapped out the entire repair dynamics for each mutant from the initial reactants to subsequent intermediates and to final products, and thus resolved each elementary reaction and determined their reaction timescales. 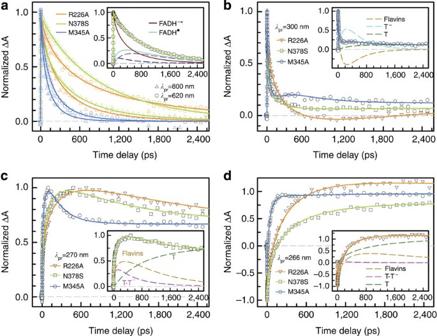Figure 2: Transient-absorption signals of three mutants probed by a wide range of wavelengths from visible to UV region at 400 nm excitation. (a) Absorption transients probed at 800 nm for detection of the excited-state flavin (FADH−*) and at 620 nm mainly for the intermediate-state flavin (FADH·). Shown in the inset is the deconvolution of the FADH−* and FADH·contributions. The latter is from two channels (dashed lines). (b–d) Absorption transients probed at (b) 300 nm, (c) 270 nm and (d) 266 nm with distinct dynamic patterns for each mutant. Shown in the insets is the deconvolution of the transient signals with detection of initial reactants, subsequent intermediates and final products for (b) M345A, (c) N378S and (d) R226A. Figure 2 shows five typical transient-absorption signals detected by a series of wavelengths from visible to UV light region for three mutants of M345A, N378S and R226A. At 800 nm, only the excited FADH − * dynamics is detected. All the dynamics in the presence of substrate follow a stretched single-exponential decay ( Fig. 2a and Supplementary Fig. 1a ), ( A , amplitude; τ , decay time constant; and β , stretched parameter), due to the modulation of ET by active-site solvation on similar timescales [11] , [12] , [13] , [19] , [20] . Using and knowing the deactivation lifetimes ( τ LT ) in nanoseconds in the absence of substrate ( Supplementary Fig. 2 and Supplementary Table 1 ), we derived the average forward ET times ( τ FET ) for six mutants ( Fig. 3a and Supplementary Table 1 ) and observed a significant change from 236 ps for the WT to 140 ps for M345A and 1,181 ps for N378C, reflecting the strong modulation of initial photoinduced processes by the active-site critical residues. These measurements are accurate and the experiments were repeated for more than four times. Given by our single-to-noise ratio, the time constants we obtained here and thereafter have an error of <10%. From these lifetimes, we obtained the first-branching quantum yields (Φ FET ) shown in Fig. 3a ( Supplementary Table 1 ). Knowing the total repair yields ( Figs 1c and 3a ), we obtained the second-branching quantum yields (Φ SP2 ) as also shown in Fig. 3a . At 620 nm, all the transient signals become slower because we also detected the intermediate radical FADH · in addition to the excited FADH − * ( Fig. 2a and Supplementary Fig. 1a ). After subtracting the excited-state FADH − * signals, we obtained the overall formation and decay dynamics of the intermediate FADH · (inset in Fig. 2a and Supplementary Fig. 1a ). The formation dynamics reflects the initial ET process of the excited FADH − * and the decay dynamics represents the electron return to the cofactor and the completion of the entire photocycle. Figure 2: Transient-absorption signals of three mutants probed by a wide range of wavelengths from visible to UV region at 400 nm excitation. ( a ) Absorption transients probed at 800 nm for detection of the excited-state flavin (FADH − *) and at 620 nm mainly for the intermediate-state flavin (FADH · ). Shown in the inset is the deconvolution of the FADH − * and FADH · contributions. The latter is from two channels (dashed lines). ( b – d ) Absorption transients probed at ( b ) 300 nm, ( c ) 270 nm and ( d ) 266 nm with distinct dynamic patterns for each mutant. Shown in the insets is the deconvolution of the transient signals with detection of initial reactants, subsequent intermediates and final products for ( b ) M345A, ( c ) N378S and ( d ) R226A. 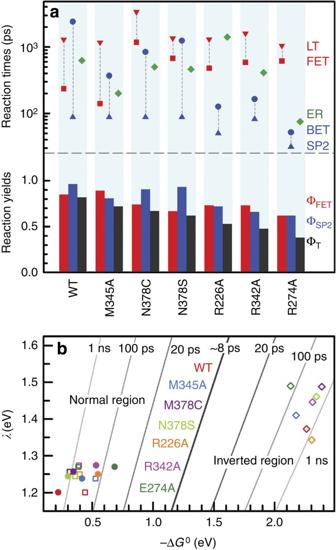Figure 3: The derived reaction times, various quantum yields and electron-transfer reorganization energies involved in DNA repair by photolyase. (a) The reaction times for five elementary reactions involved in repair. LT=deactivation lifetime; FET=forward electron transfer; BET=back electron transfer; SP2=the second C6-C6′ splitting; ER=electron return after repair. The first C5-C5′ splitting is ultrafast for all mutants within 10 ps and not shown here. The dashed lines link two sets of two competition channels responsible for the repair efficiency. Also shown are the corresponding quantum yields of ΦFETand ΦSP2for the two sets of competitions and the resulting total quantum yield of ΦT(ΦFET× ΦSP2). (b) Two-dimensional (2D) contour plot of the electron-transfer dynamics relative to free energy (ΔG0) and reorganization energy (λ) for FET (filled circle), BET (open square) and ER (open diamond) obtained in this study. The former two are in the ET normal region and the latter one is in the Marcus inverted region. Full size image Figure 3: The derived reaction times, various quantum yields and electron-transfer reorganization energies involved in DNA repair by photolyase. ( a ) The reaction times for five elementary reactions involved in repair. LT=deactivation lifetime; FET=forward electron transfer; BET=back electron transfer; SP2=the second C6-C6′ splitting; ER=electron return after repair. The first C5-C5′ splitting is ultrafast for all mutants within 10 ps and not shown here. The dashed lines link two sets of two competition channels responsible for the repair efficiency. Also shown are the corresponding quantum yields of Φ FET and Φ SP2 for the two sets of competitions and the resulting total quantum yield of Φ T (Φ FET × Φ SP2 ). ( b ) Two-dimensional (2D) contour plot of the electron-transfer dynamics relative to free energy (Δ G 0 ) and reorganization energy ( λ ) for FET (filled circle), BET (open square) and ER (open diamond) obtained in this study. The former two are in the ET normal region and the latter one is in the Marcus inverted region. Full size image Dimer splitting and repair photocycle To reveal the complete photocycle and determine how the dimer splits, we tuned our probing wavelengths to the UV region to detect thymine-related species. Figures 2b–d show three typical transients probed at 300, 270 and 266 nm with the markedly different dynamic patterns, reflecting the different contributions of various species. Knowing the flavin dynamics above and the second-branching quantum yields Φ SP2 from Φ T /Φ FET ( Fig. 3a ), with a global analysis of all transients based on the resolved repair model ( Fig. 1a , see Supplementary Note 1 for detailed analyses) [13] , we resolved the dynamics of T-T − after ultrafast C5-C5′ bond breaking ( Fig. 2c,d ), T − formation after complete dimer splitting ( Fig. 2b ) and T formation after electron return to restore the active cofactor ( Figs 2b–d ), and thus determined the sequential dynamics of the dimer splitting, the dynamics of futile back ET ( τ BET ) without repair and the electron return ( τ ER ) after successful repair ( Figs 1a and 3a ), also revealing the total intermediate FADH · decay (inset in Fig. 2a ) from the two contributions of the branched back ET and repair channels (dashed lines). Reaction timescales and repair efficiency All the dynamics and timescales of the elementary reactions are shown in Fig. 3a ( Supplementary Table 1 ). To reach high repair efficiency Φ T , both the first-branching Φ FET and second-branching Φ SP2 need to be as large as possible, that is, the FET and dimer splitting should be as fast as possible, and the deactivation process and futile BET as slow as possible. Clearly, mutations either at the cofactor side or the substrate side significantly modulate the three ET reactions of FET, BET and ER. For the dimer splitting, the first C5-C5′ bond breakage is ultrafast in <10 ps [13] , [21] , [22] for all the mutants but the critical second C6-C6′ cleavage is modulated by the mutations around the substrate. Specifically, for M345A, the FET (140 ps) is faster than that of the WT (236 ps), leading to an even larger Φ FET of 0.89. All other mutants have slower FET dynamics, resulting in a smaller Φ FET of 0.74–0.62 than the WT (0.85). For the competition between the dimer splitting and futile BET, all the mutants have faster futile BET dynamics. Although the mutants of R226A and E274A have faster C6-C6′ splitting dynamics, their BET also becomes faster. Finally, all mutations result in a smaller Φ SP2 of 0.93–0.62. For M345A, although the initial photoinduced reaction is even faster than the WT with the largest Φ FET , the smaller Φ SP2 dominates and therefore leads to a lower Φ T . Thus, unlike other biological photochemical systems, the initial photoinduced process in photolyase does not have to be ultrafast and the main determinant of overall high repair efficiency. For all other five mutants, both the smaller Φ FET and Φ SP2 lead to a lower total repair efficiency Φ T of 0.67–0.38 ( Fig. 3a ). The significant modulation of the three ET reactions by the mutations provides insight to contributing factors to overall repair efficiency. The deactivation process and the second C6-C6′ bond splitting, except for N378C and E274A, respectively, are quite similar ( Fig. 3a ). Thus, the interplay between FET and BET is critical to modulating the repair yield. The WT enzyme has the slowest BET (2.4 ns) and very faster FET (236 ps), leading to the highest repair yield. For all the mutants, the FET dynamics with the exception of M345A become slower and all the BET processes become faster, and thus unfavourable for repair. To understand these changes, we evaluated these ET reactions using the Marcus ET theory to estimate the driving forces (−Δ G 0 ) and reorganization energies ( λ ) [23] , [24] , [25] , [26] for each form of the enzyme (see Supplementary Note 2 ). Figure 3c shows the derived results of Δ G 0 and λ for the FET, BET and ER. The FET is in the Marcus normal region (−Δ G 0 ≤ λ ). The BET is a dissociative ET process [21] . For the C5-C5′ cleavage, the BET has a small driving force and is in the normal region again, due to a high energy of the neutral intermediate T-T after charge recombination [21] , [25] . The ER after repair is in the Marcus inverted region (−Δ G 0 ≥ λ ). The mutations considerably alter not only the free energy changes, that is, the reduction potentials of the cofactor or the substrate, but also the reorganization energies [20] , [25] , [26] and thus significantly modulate all three ET reactions. The derived large reorganization energies mainly come from the contributions of the different structural distortions of FADH − and FADH · (refs 25 , 27 ). The obtained changes of driving forces and reorganization energies for three ET reactions by mutations are basically correlated with the local structural and chemical properties (for details, see Supplementary Note 3 : influence of the mutations on the electron transfer reactions and the dimer splitting). 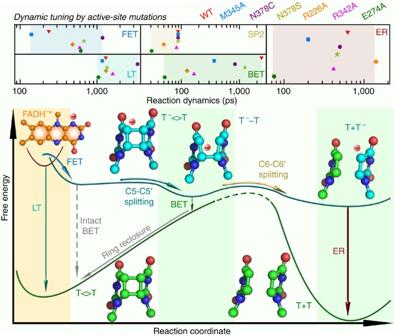Figure 4: Reaction free-energy profile along reaction coordinate for complex enzymatic DNA repair. Six elementary reaction steps (solid lines) with the structures of the excited cofactor flavin (orange) and all thymine-related intermediates (blue) and products (green). The relative energy between each state is mainly determined from our dynamic measurements. The seventh elementary step of intact BET (dashed line) is slow and does not happen in the entire repair due to the ultrafast C5-C5′ splitting. The reactions times are displayed at the top to show direct modulation of five elementary steps by the six mutations with the wild type included for comparison. Figure 4 shows the entire energy profile of the enzymatic repair along the reaction coordinate with at least six fundamental steps including the excited-state deactivation, three ET elementary reactions and two sequential bond breaking and making processes. To maximize the repair efficiency, the enzyme has a relatively rigid active site, structurally and electrostatically, to avoid the ultrafast deactivation from the butterfly bending motion and lengthen the excited-state lifetime [27] , [28] , and a favourable redox environment to lead to an appropriate FET, not too slow so as to result in lower Φ FET and not too fast so as to cause faster BET with a lower Φ SP2 . After charge separation, the reaction proceeds to the ultrafast C5-C5′ bond splitting, thus eliminating the first intact charge-recombination channel to the original ground state without the dimer splitting. After the first C5-C5′ bond breaking, the reaction encounters a small barrier for the second C6-C6′ bond splitting and the reaction bifurcates. The second charge-recombination channel that leads to the closure of the dimer ring again competes with the productive second C6-C6′ bond cleavage, leading to a loss of the repair yield. The redox property at the active site is synergistically optimized to balance the FET and BET processes relative to the excited-state deactivation and the dimer splitting, respectively, to achieve the maximum outcome. After the complete dimer splitting, the third charge-recombination channel, the elector return to restore the active flavin cofactor and complete the repair photocycle, should not be too slow to avoid new damage of repaired DNA by the extra electron [29] . Any mutation as studied here that modulates the active-site reduction potentials and ET reorganization energies always breaks the dedicated synergy of the optimization for the main four elementary reactions in two competitions, and thus leads to lower repair efficiency than the WT enzyme. Figure 4: Reaction free-energy profile along reaction coordinate for complex enzymatic DNA repair. Six elementary reaction steps (solid lines) with the structures of the excited cofactor flavin (orange) and all thymine-related intermediates (blue) and products (green). The relative energy between each state is mainly determined from our dynamic measurements. The seventh elementary step of intact BET (dashed line) is slow and does not happen in the entire repair due to the ultrafast C5-C5′ splitting. The reactions times are displayed at the top to show direct modulation of five elementary steps by the six mutations with the wild type included for comparison. Full size image Preparation of photolyase and mutants The purification of E. coli photolyase without the antenna cofactor has been reported elsewhere [30] , [31] . For mutant enzyme studies, we mutated a series of key residues at the active site (R226A, E274A, N341A, R342A, M345A, N378C and N378S) using QuikChange II XL kit (Stratagene) based on the plasmid of wild-type enzyme. All mutated plasmids were sequenced to confirm the mutations and ensure the absence of secondary mutations. After the standard purification, all mutant proteins were obtained with stoichiometric flavin except N341A that lacks the FAD cofactor. In femtosecond spectroscopic studies, 100 μM of enzyme (or 50 μM in experiments with probe wavelengths of shorter than 300 nm) was used in a reaction buffer containing 100 mM NaCl, 50 mM Tris-HCl at pH 7.5, 20 mM dithiothreitol, 1 mM EDTA and 50% (v/v) glycerol. Preparation of cyclobutane thymine dimer substrate We prepared the cyclobutane thymine dimer (T<>T) substrate from oligo(dT) 15 as described elsewhere with some modification [32] . In brief, we dissolved 3 mg oligo(dT) 15 (synthesized by Integrated DNA Technologies) in 1 ml 15% aqueous acetone (v/v). The argon-purged DNA solutions were irradiated over ice with a 302-nm UVB lamp (General Electric) at a 2-cm distance for 50–70 min. T<>T formation was monitored by decreases in absorbance at 260 nm. In the final products, there are about five T<>T dimers in each strand of oligo(dT) 15 . The concentration of the oligosubstrates used in the femtosecond studies is 3 mM (or 1.5 mM in experiments with probe wavelengths of shorter than 300 nm). Enzyme activities The enzyme activities of the wild-type and mutant photolyases were quantitatively measured. Procedures for determination of dissociation constants and relative quantum yields of the mutants were described before [13] , [25] . For each mutant, a set of mixtures of 1 μM enzyme with different concentrations (111, 333, 500 and 1,000 μM) of T<>T-containing oligo(dT) 15 substrate was prepared. These samples in cuvettes were irradiated at the room temperature using white-light lamp (General Electric) at the same distance of 6 cm. The absorption spectra of each mixture were recorded at a series of illumination times. The increased absorbance around 266 nm is a measure of the formation of thymine bases. Figure 1c shows typical steady–state repair measurements for the wild-type and six mutant photolyases. For each enzyme–substrate binding complex (ES), the absorbance change at 266 nm was plotted vs illumination times, and the slope is directly proportional to the binding complex concentration ([ES]) and the repair efficiency of the enzyme. Considering that some part of enzymes is not bound with substrates, the dissociation constants ( K d ) for each mutant need to be carefully determined. The binding complex percentage ([ES]/[E]) for each enzyme is plotted against different substrate concentrations ( Supplementary Fig. 3 ), and the dissociation constants were fit by the equation [ES]/[E]=[S]/([S]+ K d ). The derived dissociation constants are 8.3 × 10 −6 , 1.2 × 10 −5 , 1.4 × 10 −5 , 2.0 × 10 −4 , 5.0 × 10 −5 , 2.4 × 10 −5 and 1.2 × 10 −5 M for wild type (WT), E274A, R226A, R342A, M345A, N378C and N378S, respectively. R342A has the largest dissociation constant, which is consistent with the crystal structure that R342 has many H-bonds with the water network at the binding site and the direct interaction with the phosphate of DNA backbone [18] . The repair quantum yields for the mutants were calculated by comparing the slopes of mutants with that of WT ( Fig. 1c ), taking account of the enzyme–substrate concentration extracted from the dissociation constants. Knowing the repair quantum yield of the WT to be 0.82 (refs 8 , 13 , 25 , 33 ), the repair quantum yields for the mutants were obtained ( Supplementary Table 1 ). Femtosecond-resolved spectroscopy All the femtosecond-resolved measurements were carried out using transient absorption methods. The laser experimental layout and procedure have been detailed elsewhere [34] , [35] . One-mm quartz cuvettes (Starna) were used as the sample cell in experiments with the probe wavelengths of shorter than 300 nm, while 5-mm cuvettes were used for other experiments. The samples were stirred during irradiation to avoid heating and photobleaching. All experiments in the femtosecond-resolved measurements were carried out under anaerobic conditions. How to cite this article: Tan, C. et al . The molecular origin of high DNA-repair efficiency by photolyase. Nat. Commun. 6:7302 doi: 10.1038/ncomms8302 (2015).